Protein grafting of p53TAD onto a leucine zipper scaffold generates a potent HDM dual inhibitor Reactivation of the p53 pathway by a potential therapeutic antagonist, which inhibits HDM2 and HDMX, is an attractive strategy for drug development in oncology. Developing blockers towards conserved hydrophobic pockets of both HDMs has mainly focused on small synthetic compounds; however, this approach has proved challenging. Here we describe an approach to generate a potent HDM dual inhibitor, p53LZ2, by rational protein grafting of the p53 transactivation domain onto a homodimeric leucine zipper. p53LZ2 shows tight binding affinity to both HDMs compared with wild-type p53 in vitro . X-ray crystallographic, comparative modelling and small-angle X-ray scattering studies of p53LZ2-HDM complexes show butterfly-shaped structures. A cell-permeable TAT-p53LZ2 effectively inhibits the cancer cell growth in wild-type but not mutant p53 by arresting cell cycle and inducing apoptosis in vitro . Thus, p53LZ2, designed by rational grafting, shows a potential therapeutic approach against cancer. The cellular level of p53 in unstressed normal cells is tightly controlled by an auto-regulatory feedback loop that regulates the activity of p53 protein and the expression level of a specific gene encoding a potent p53-negative regulator HDM2 (ref. 1 ). The transcription factor p53 binds to the E3 ubiquitin ligase HDM2 gene and the elevated intracellular level of HDM2 protein in turn decreases the endogenous p53 by a direct interaction between the N-terminal domains of both proteins resulting in proteasome-mediated degradation of poly-ubiquitinated p53 (ref. 2 ). While several previously identified E3 ubiquitin ligases out of HDM2 (for example, Pirh2, COP1 and ARF-BP1) [3] , [4] , [5] target p53 for ubiquitin-mediated degradation, there is no direct evidence that any of these ligases can replace HDM2 to regulate p53 stability in cancer cells [6] . On the other hand, a close relative of HDM2, HDMX (also called HDM4), is known to control p53 status in cancer cells through a direct interaction that neutralizes the transcriptional activation potency of the transactivation domain of endogenous p53 (hereafter p53TAD) in a similar way as observed in the p53-HDM2 interaction. HDMX per se does not act as the E3 ubiquitin ligase of p53, but rather enhances HDM2 ligase activity mediated by the C-terminal RING–RING interaction between HDM2 and HDMX, albeit the function of HDM2-HDMX hetero-dimerization has not been completely clarified yet [7] , [8] , [9] , [10] . Interestingly, HDM2 is not only a bona fide E3 ubiquitin ligase for p53 but also ubiquitinates HDMX [11] . Thus, HDM2 serves as a key regulator that orchestrates HDMX stability as well as p53 activity in vivo . In terms of a therapeutic point of view, tumour suppressor p53 is a potent anti-proliferative, anti-apoptotic guardian molecule that induces cell cycle arrest, apoptosis, autophagy and senescence in cancer cells [12] . Almost 11 million patients suffering from various cancer types worldwide are known to bear wild-type p53 in tumours [13] . Thus, reactivation of the p53 pathway by displacing the negative regulator HDM2 and/or its homologue HDMX from endogenous wild-type p53 in cancer cells has long been considered an important therapeutic strategy in oncology. Accordingly, numerous innovative efforts from academic laboratories as well as pharmaceutical industries have been focused on developing synthetic compounds, peptidomimetics or miniature protein antagonists of the p53–HDM2 (and HDMX) interaction [14] , [15] , [16] , [17] , [18] , [19] , [20] , [21] , [22] , [23] . Among them, the first reported HDM2-specific inhibitor Nutlin-3, which mimics three essential hydrophobic residues of wild-type p53 (F19, W23 and L26; human p53 numbering) required for HDM2 recognition, demonstrated that this small compound disrupting the p53–HDM2 interaction recovered p53 function and resensitized cancer cells to apoptosis in vitro and in vivo [18] . In fact, the p53TAD is largely unstructured under physiological conditions, while transforming into an α-helical conformation when interacting with target proteins in the presence of binding partners such as RPA and HDMs [24] . Recent studies of a stapled p53-based peptide, which contains a chemical hydrocarbon crosslink within a synthetic peptide (stapling), demonstrated that the p53 peptidomimetic restored the intrinsic α-helix-forming tendency of p53TAD and conferred the intracellular protease resistance [25] , [26] , [27] . Such seminal structural insights into the stabilized α-helix (SAH) of p53 inspired us to challenge this attractive target in oncology and design a new molecular entity of a p53TAD mimetic. Here we describe a new approach in generating a potent HDM2 and HDMX dual antagonist by rational protein grafting of p53TAD onto the GCN4 leucine zipper domain (hereafter GCN4LZ), a well-known homodimeric α-helical scaffold having a completely helical structure extensively stabilized by the intra-chain salt bridges as well as the inter-chain hydrophobic interactions [28] , [29] . By transferring the three key hydrophobic residues of p53TAD, F14, W18 and L21 (new numbering in this study, see Fig. 1a ) onto the ideal positions of each helix in the GCN4LZ homodimer and also adding two more substitutions, G10 and S15 (new numbering), which further fine-tune the binding affinity of a designed p53TAD mimetic against HDM2 and HDMX, we generate a potent dual inhibitor with high binding affinity against both HDMs in comparison with wild-type p53 in vitro . We also report the X-ray crystallographic, comparative protein structure modelling and small-angle X-ray scattering (SAXS) studies of coiled-coil architecture of the GCN4LZ-driven p53TAD mimetic (hereafter p53LZ) and its complex with the N-terminal domain of either HDM2 or HDMX. Further biochemical and cell-based studies exhibit an impressive on-target biological efficacy of a cell penetrating p53LZ (TAT-p53LZ2) in various cancer cell lines expressing wild-type but not mutant p53. Reactivation of the p53 pathway by our designed p53LZ2 shows a potential therapeutic possibility against cancer and provides a framework to advance the development of peptide-based biologics in drug discovery technology. 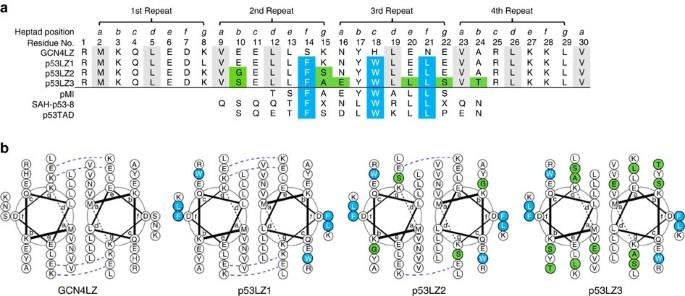Figure 1: p53LZ design concept. (a) Sequence alignment of GCN4LZ and designed p53LZs. Two different peptides showing high affinities against HDM2 and HDMX (pMI and SAH-p53-8) together with naturally occurring WT p53 (p53TAD) aligned to GCN4LZ and designed p53LZs. Three key hydrophobic residues, F, W and L, are highlighted in blue. Additional substitutions of amino acids in p53LZ1, p53LZ2 and p53LZ3 are shown in green. Each heptad repeat is marked at the top of GCN4LZ sequence. (b) Helical wheel representations of GCN4LZ and grafted p53LZs. Figure 1: p53LZ design concept. ( a ) Sequence alignment of GCN4LZ and designed p53LZs. Two different peptides showing high affinities against HDM2 and HDMX (pMI and SAH-p53-8) together with naturally occurring WT p53 (p53TAD) aligned to GCN4LZ and designed p53LZs. Three key hydrophobic residues, F, W and L, are highlighted in blue. Additional substitutions of amino acids in p53LZ1, p53LZ2 and p53LZ3 are shown in green. Each heptad repeat is marked at the top of GCN4LZ sequence. ( b ) Helical wheel representations of GCN4LZ and grafted p53LZs. Full size image Rational protein grafting of p53TAD onto the GCN4LZ The GCN4LZ encompassing 30 residues shows the characteristic seven-residue (heptad) repeat (a–f) n , where hydrophobic or charged residues are positioned at the (a, d) and (e, g) slots, respectively ( Fig. 1a ). The GCN4LZ core, which consists of (a, d) and (e, g) positions, is not easily accessible by its binding partners, whereas the (c, h, f) side-chains protruding from the GCN4LZ surface can be considered as desired areas for p53TAD grafting because of the large solvent accessible area of homodimeric GCN4LZ (PDB ID 2ZTA, ~5,101 Å 2 ). Therefore, these latter residues were primarily tested for the grafting of p53TAD onto the GCN4LZ ( Fig. 1b ). The side-chain orientations of the three key hydrophobic residues, F19, W23 and L26 (human p53 numbering), of p53 directs towards the conserved hydrophobic pockets on HDM2 and HDMX, showing complementarity to the HDM pockets [30] , [31] . We chose (c, f) positions of the 2nd and 3rd heptad repeats (a9–g22) to graft F, W and L residues onto the GCN4LZ because disturbing the 1st and 4th (trigger site of the GCN4LZ) repeats decreases the overall protein stability more than other repeats ( Fig. 1b ). These grafted p53TAD mimetics, which are named p53LZ1, p53LZ2 and p53LZ3, contain 3, 5 and 9 mutation points, respectively. p53LZ1 has the simplest amino-acid substitution on the GCN4LZ, whereas p53LZ3, bearing more a complicated substitution, is designed to be more similar to the pMI sequence (TSFAEYWALLS), one of the previously identified high-affinity peptides against the HDM2 and HDMX [17] . Two additional changes onto the p53LZ2, E10G and K15S, in addition to the three key hydrophobic residues, were carefully identified to strengthen the protein–protein interaction between the designed p53LZ and HDM proteins based on the structural analysis by comparative structure modelling. We also calculated the free energy of binding of the designed p53LZ to the HDM2 N-terminal domain by using the available X-ray structures (PDB ID 1YCR and 2ZTA) and GROMACS [32] software to simulate the possible binding mode of each complex. Molecular dynamic simulations coupled with MM/PBSA (Molecular Mechanics/Poisson–Boltzmann Surface Area) approach were carried out for 60 ns. The calculated binding energy (Δ G comp ) of the p53LZ2–HDM2 complex exhibited the lowest value of −41.5 kJ mol −1 , whereas the HDM2 N-terminal domain in complex with either p53LZ1 or p53LZ3 revealed a relatively higher binding energy (−9.0 or 6.9 kJ mol −1 ) compared with the p53LZ2-HDM2 complex, suggesting that the E10G and K15S substitutions in the p53LZ2 sequence may contribute to the higher affinity binding ( Supplementary Table 1 ). Two mutations, E20L and E22S, in p53LZ3, which originally interacts with K94 and K51 of HDM2, respectively, likely impair the p53LZ3-HDM2 interaction by disrupting electrostatic interactions between both proteins, revealing significant differences of the calculated coulombic (Δ G coul =710.8 kJ mol −1 ) and polar solvation (Δ G ps =−262.6 kJ mol −1 ) terms, relative to those of p53LZ1 and p53LZ2 ( Supplementary Fig. 1 and Supplementary Table 1 ). Characterization of HDM2 and HDMX interaction with p53LZ To assess the binding of HDM2 and HDMX to p53LZ in vitro , we expressed and purified recombinant GST-p53LZ proteins (p53LZ1, p53LZ2 and p53LZ3) and N-terminal domains of His6-HDM2 and His6-HDMX corresponding to residues 1–125 and 1–132, respectively (hereafter HDM2NTD and HDMXNTD) and then performed an in vitro GST pull-down assay ( Fig. 2a ). GST-p53LZ1 and GST-p53LZ2 effectively pulled down both HDM2NTD and HDMXNTD, whereas GST and GST-p53LZ3 did not show a relevant interaction with either HDM2NTD or HDMXNTD, demonstrating a direct physical interaction of HDM2 and HDMX with the designed p53LZ1 and p53LZ2 in vitro . Apparently, GST-p53LZ2, compared with GST-p53LZ1 binds preferentially to both HDM2NTD and HDMXNTD, suggesting that the two additional substitutions in the p53LZ2, E10G and K15S contribute to a tight interaction with HDM2 and HDMX ( Fig. 3 ). Further binding studies with analytical size-exclusion chromatographic (SEC) analysis demonstrated a direct interaction between p53LZ2 and both HDM N-terminal domains, revealing co-migration of p53LZ2 and its binding partner in gel filtration ( Fig. 2b ). To precisely determine the stoichiometry between p53LZ2 and both HDM2NTD and HDMXNTD, we used multi-angle light scattering (MALS) analysis in conjunction with refractive index, which measures molecular mass independent of its molecular shape. The result indicates the existence of a homogeneous species for p53LZ2–HDM2NTD or p53LZ2–HDMXNTD heterotetrameric complex in solution with a corresponding molecular mass of 40.2 or 41.6 kDa, respectively, confirming a 1:2 stoichiometry between p53LZ2 homodimer and both HDM N-terminal domains ( Fig. 2c ). 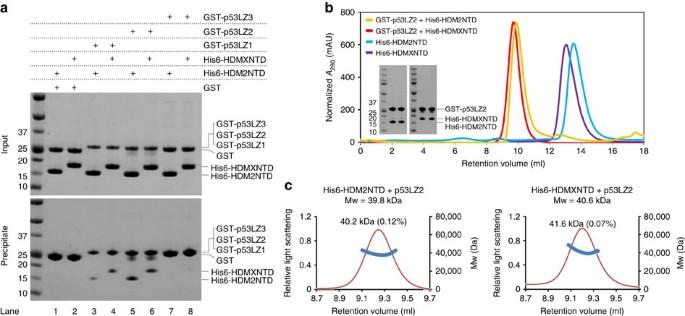Figure 2: p53LZ1 and p53LZ2 interact with both HDM2 and HDMXin vitro. (a)In vitroGST pull-down assay of designed p53LZs against both HDM2 and HDMX N-terminal domains (HDM2NTD and HDMXNTD). GST or GST-tagged proteins were incubated with HDM2NTD or HDMXNTD and then the protein mixtures were precipitated with glutathione resin after washing to remove unbound proteins. (b) Gel filtration analysis on GST-p53LZ2 in the absence and presence of HDM2NTD or HDMXNTD. The retention volumes and SDS–PAGE results are indicated. (c) Multi-angle light scattering (MALS) measurement of p53LZ2 bound to HDM2NTD or HDMXNTD showing the relative light scattering signal as a function of elution volume. The measured molecular mass of each peak is shown in blue. Figure 2: p53LZ1 and p53LZ2 interact with both HDM2 and HDMX in vitro. ( a ) In vitro GST pull-down assay of designed p53LZs against both HDM2 and HDMX N-terminal domains (HDM2NTD and HDMXNTD). GST or GST-tagged proteins were incubated with HDM2NTD or HDMXNTD and then the protein mixtures were precipitated with glutathione resin after washing to remove unbound proteins. ( b ) Gel filtration analysis on GST-p53LZ2 in the absence and presence of HDM2NTD or HDMXNTD. The retention volumes and SDS–PAGE results are indicated. ( c ) Multi-angle light scattering (MALS) measurement of p53LZ2 bound to HDM2NTD or HDMXNTD showing the relative light scattering signal as a function of elution volume. The measured molecular mass of each peak is shown in blue. 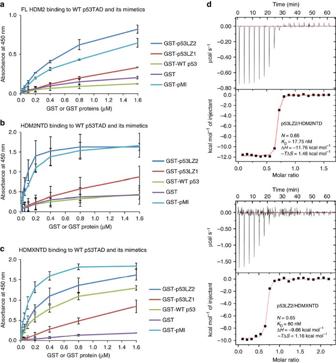Figure 3: p53LZ2 exhibits high-affinity binding to both HDM2 and HDMX, relative to WT p53in vitro. GST or GST proteins were used in ELISA assays of (a) MBP-FL HDM2, (b) MBP-HDM2NTD and (c) MBP-HDMXNTD binding. GST-p53LZ2 harbouring five grafted residues, G10, F14, S15, W18 and L21, showed significantly higher binding affinities to HDM2 and HDMX in comparison with WT p53TAD (residues 1–72) and GST-p53LZ1. All data are presented as mean±s.d. of three independent experiments. (d) ITC titration and fitting curves for p53LZ2 binding to HDM2NTD or HDMXNTD. The numbers show the fitting of the data, withN(stoichiometry),KD(dissociation constant), ΔH(enthalpy change) and −TΔS(entropy change). Full size image Figure 3: p53LZ2 exhibits high-affinity binding to both HDM2 and HDMX, relative to WT p53 in vitro. GST or GST proteins were used in ELISA assays of ( a ) MBP-FL HDM2, ( b ) MBP-HDM2NTD and ( c ) MBP-HDMXNTD binding. GST-p53LZ2 harbouring five grafted residues, G10, F14, S15, W18 and L21, showed significantly higher binding affinities to HDM2 and HDMX in comparison with WT p53TAD (residues 1–72) and GST-p53LZ1. All data are presented as mean±s.d. of three independent experiments. ( d ) ITC titration and fitting curves for p53LZ2 binding to HDM2NTD or HDMXNTD. The numbers show the fitting of the data, with N (stoichiometry), K D (dissociation constant), Δ H (enthalpy change) and − T Δ S (entropy change). Full size image In vitro binding of wild-type p53 and its mimetics to HDMs To further investigate the designed p53LZs in interaction with either HDM2 or HDMX, we assessed the binding of MBP-fused HDM proteins, full-length (FL) HDM2, HDM2NTD and HDMXNTD to GST, GST wild-type (WT) p53TAD, GST-p53LZ1 and GST-p53LZ2, purified from E. coli in ELISA. In addition, a well-known high-affinity variant of p53TAD (pMI) [17] previously identified by phage display was also produced as GST-tagged proteins to compare its relative binding affinity to HDM2 and HDMX. The ELISA plate coated with MBP-FL HDM2, MBP-HDM2NTD or MBP-HDMXNTD was incubated with increased amounts of GST or GST-fused proteins. A horseradish peroxidase-conjugated anti-GST antibody was used to detect the bound protein. p53LZ2, harbouring a total of five grafted residues, bound preferentially to both HDM2 and HDMX compared with others, suggesting that the two more grafting (G10 and S15) in addition to the essential hydrophobic residues (F14, W18 and L21) onto the GCN4LZ is critical for tight interaction with both HDM proteins ( Fig. 3a–c ). Furthermore, the quantitative ELISA studies revealed a relatively similar binding of GST-p53LZ2 and GST-pMI to both HDM2 and HDMX. To quantify the target-binding strength of grafted p53LZ2 in vitro , we measured the direct binding affinity of p53LZ2 to HDM2NTD and HDMXNTD using isothermal titration calorimetry (ITC) ( Fig. 3d ). p53LZ2 strongly bound to HDM2NTD ( K D =18 nM), exceeding a previously reported value of WT p53TAD for HDM2NTD ( K D =61.3 nM, measured in PBS containing 0.1 mM TCEP and 0.01% NaN 3 ) [17] , whereas the p53LZ2 homodimer exhibited a moderately higher affinity for HDMXNTD ( K D =80 nM) in comparison to a previously determined ITC data ( K D =202 nM, measured in PBS containing 0.1 mM TCEP and 0.01% NaN 3 ) [17] . The enthalpy–entropy compensation in both cases was revealed by favourable enthalpy (Δ H ) and unfavourable entropy (− T Δ S ) changes, which contribute to a high-affinity binding of p53LZ2 to both HDM N-terminal domains. In addition, the binding stoichiometry ( N ) determined by the ITC analysis further supports that homodimeric p53LZ2 preferentially interacts with both HDM proteins in 1:2 complexes ( Fig. 3d ). Structural analysis of HDM2 and HDMX recognition by p53LZ2 Next, we performed three distinct experiments to investigate the structural mechanism of HDM2 and HDMX recognition by p53LZ2. First, we conducted circular dichroism (CD) experiments to evaluate the structural impact of protein grafting onto the GCN4LZ. The recombinant p53LZ2 and its parent molecule GCN4LZ displayed highly α-helical conformations (>90% helicity) in physiological pH and almost identical T m values (~63 °C), suggesting that the protein grafting strategy of p53TAD onto this homodimeric scaffold to facilitate target binding did not alter the overall structural integrity of GCN4LZ ( Supplementary Fig. 2 ). Second, we determined a high-resolution (1.2 Å) crystal structure of p53LZ2 harbouring substitution in five residues on the GCN4LZ ( Table 1 ). The initial electron density map corresponding to homodimeric parallel coiled-coil architecture of the grafted p53LZ2 was readily generated in high quality by molecular replacement method using the GCN4LZ as search model ( Fig. 4a and Supplementary Fig. 3 ). The refined high-resolution structure of p53LZ2 is a twisted elliptical cylinder protruding the key HDM binding residues F14, W18 and L21 from the main-chains of both helices. Furthermore, two parallel α-helices are associated with tightly packed conformations stabilized by the inter-chain salt bridges, R1–E6, S15–N16, N16–N16 and E22–K27 as well as the extensive inter-chain hydrophobic interactions, L5–L5, V9–V9, L12–L12, L12–L13, L19–L19, V23–V23, L26–L26, L29–V30 and V30–V30. Interestingly, K15S mutation in the p53LZ2 likely compensated the loss of K15–E20 interaction between the two helices of GCN4LZ ( Fig. 1b ) by creating a new inter-chain S15–N16 interaction. To understand the HDM2 and HDMX recognition by p53LZ2 homodimer, we generated a complex structure for p53LZ2 bound to HDM2NTD or HDMXNTD using HADDOCK [33] . The sophisticated structural superposition of WT p53TAD-HDM2 or HDMX and the HADDOCK structure were also conducted to evaluate protein–protein docking. The key HDM-binding residues, F14, W18 and L21, of p53LZ2 were situated along one face of each α-helix and well positioned into the three hydrophobic pockets of both HDM2NTD and HDMXNTD, as similarly observed in the wild-type complexes ( Fig. 4b,c ). In contrast, E10G and K15S substitutions of p53LZ2 contributed towards reducing possible steric clash between adjacent side-chains of GCN4LZ and HDM proteins (for example, GCN4LZ E10—HDM2 Q69, Q72 and GCN4LZ K15—HDM2 M62) and optimizing spatial arrangement in p53LZ2-HDM interaction for enhanced binding. The p53LZ2–HDM2 interaction is further reinforced by numerous electrostatic interactions between both proteins for example, p53LZ2 K3, E6, D7, E20, K27 and HDM2 E69, K70, R65, K94, E52, respectively ( Supplementary Fig. 4 ), supporting the notion that a high-affinity binding of p53LZ2 to HDMs is likely attributed to large binding areas through the N-terminal and C-terminal segments of p53LZ2 in part. As a third experiment, given the available crystal structures and possible protein complex models, we co-purified homodimeric p53LZ2 in complex with either HDM2NTD or HDMXNTD from E. coli and further investigated the resulting protein complexes using SAXS analysis [34] , [35] , [36] . All SAXS measurements of the p53LZ2–HDM complexes, in PBS buffer, were done in triplicate exposures and analysed to calculate the final composite scattering curves ( Fig. 4d , left). By the Guinier analysis of the SAXS scattering curves, we confirmed the absence of protein aggregation and further processed the data ( Supplementary Fig. 5 ). The maximum diameter ( D max ) from the pair distance distribution function p ( r ) and the radius-of-gyration R g of p53LZ2–HDM2NTD complex are ~60 and ~22 Å, respectively ( Fig. 4d , right). The ab initio reconstitution of p53LZ2 in complex with either HDM2NTD or HDMXNTD using GASBOR [37] represents the butterfly-shaped SAXS envelope displaying pseudo twofold symmetry ( Fig. 4e , Supplementary Figs 6 and 7 ). These reproducible envelopes show a good correlation between experimental and calculated scattering patterns (sqrt( χ )=1.347 (p53LZ2–HDM2NTD) and 1.554 (p53LZ2–HDMXNTD)). Finally, superposition of the HADDOCK structures of p53LZ2–HDM complexes onto the corresponding SAXS envelopes reveals almost perfect spatial arrangement of the two HDM2NTD or HDMXNTD wings relative to the central p53LZ2 body ( χ 2 =1.2 and χ 2 free =2.8 for p53LZ2–HDM2NTD complex, χ 2 =1.5 and χ 2 free =3.3 for p53LZ2–HDMXNTD complex) further supporting the 1:2 p53LZ2–HDM complexes in solution ( Fig. 4e and Supplementary Fig. 6 ). Table 1 Data collection and refinement statistics. 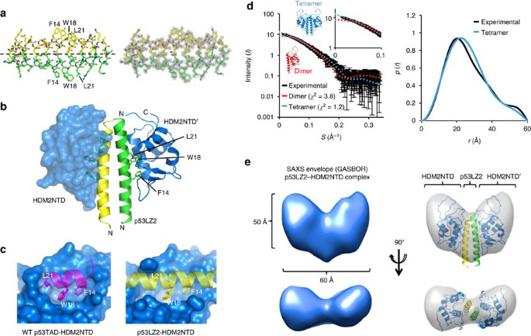Figure 4: Structural studies of p53LZ2 homodimer and its complex with HDM2NTD. (a) Overall structure of p53LZ2 homodimer at 1.2 Å (left). Three key hydrophobic residues, F14, W18 and L21, are indicated. Twofold axis of the coiled-coil is shown by dotted line. A 2Fo−Fcmap contoured at 1.0σis superimposed with p53LZ2 (right). (b) HADDOCK-based quaternary structure of p53LZ2-HDM2NTD complex. HDM2NTD molecules (marine) bound to p53LZ2 homodimer (green and yellow) are represented as surface or cartoon. Essential hydrophobic residues, F14, W18 and L21, for recognizing HDM2NTD are shown as stick. (c) Structural comparison in HDM2 binding between WT p53TAD and p53LZ2. Close-up view of the hydrophobic pockets of HDM2 (marine) for the amino acid triad, F, W and L of WT p53TAD (magenta) and p53LZ2 (yellow) are shown as surface. (d) Experimental SAXS scattering curve (black, s.e.) plotted versus the theoretical CRYSOL calculations for the dimer (red dots) and tetramer (blue dots), and normalized distribution function of p53LZ2–HDM2NTD quaternary complex are shown on the left and right, respectively. An expanded plot of the low-angle data (0<S<0.1) is shown in the top right insert (left). (e) HADDOCK-based structure, represented as a cartoon, was fitted into the SAXS envelope (blue) with dimensions. Full size table Figure 4: Structural studies of p53LZ2 homodimer and its complex with HDM2NTD. ( a ) Overall structure of p53LZ2 homodimer at 1.2 Å (left). Three key hydrophobic residues, F14, W18 and L21, are indicated. Twofold axis of the coiled-coil is shown by dotted line. A 2 F o − F c map contoured at 1.0 σ is superimposed with p53LZ2 (right). ( b ) HADDOCK-based quaternary structure of p53LZ2-HDM2NTD complex. HDM2NTD molecules (marine) bound to p53LZ2 homodimer (green and yellow) are represented as surface or cartoon. Essential hydrophobic residues, F14, W18 and L21, for recognizing HDM2NTD are shown as stick. ( c ) Structural comparison in HDM2 binding between WT p53TAD and p53LZ2. Close-up view of the hydrophobic pockets of HDM2 (marine) for the amino acid triad, F, W and L of WT p53TAD (magenta) and p53LZ2 (yellow) are shown as surface. ( d ) Experimental SAXS scattering curve (black, s.e.) plotted versus the theoretical CRYSOL calculations for the dimer (red dots) and tetramer (blue dots), and normalized distribution function of p53LZ2–HDM2NTD quaternary complex are shown on the left and right, respectively. An expanded plot of the low-angle data (0< S <0.1) is shown in the top right insert (left). ( e ) HADDOCK-based structure, represented as a cartoon, was fitted into the SAXS envelope (blue) with dimensions. Full size image p53LZ targets endogenous HDM2 and HDMX The protein transduction strategy using the positively charged cell-penetrating peptide transactivator of transcription (TAT) was applied to increase the cell permeability of designed p53LZ2, thereby overcoming the membrane barrier by endocytosis and/or direct penetration into cells [38] . To investigate the ability of p53LZ2 to target endogenous HDM2 and HDMX, we first produced the cell-permeable TAT-p53LZ2 to high purity from E. coli and then conducted immunoprecipitation studies in MCF7 (human breast carcinoma) cells. After 6 h incubation of cells treated with 10 μM of each LZ molecule (His-tagged TAT-p53LZ2 or His-tagged TAT-GCN4LZ), the cell lysates were prepared and subjected to Ni-NTA pull-down assay, followed by HDM2 and HDMX western blot analysis. The intracellular HDM2 and HDMX specifically co-precipitated with TAT-p53LZ2 but not with its non-functional equivalent TAT-GCN4LZ ( Fig. 5a ). To further evaluate the cell-penetrating TAT-p53LZ2-mediated inhibition of p53 binding by both HDM proteins in cells, we treated MCF7 with 10 μM of each LZ (TAT-p53LZ2 or TAT-GCN4LZ) for 6 h and subsequently determined the amount of endogenous HDM2 or HDMX associated with p53 in cell lysates by immunoprecipitation and western blot analysis. Our data clearly confirmed that the TAT-p53LZ2 transferred across the cell membrane induced a substantial depletion of both HDM proteins bound to the intracellular p53 in cell lysates compared with those of TAT-GCN4LZ ( Fig. 5b ). Taken together, these data demonstrate that TAT-p53LZ2 targets both HDM2 and HDMX in situ , showing the expandability of our research scope to the cellular level. 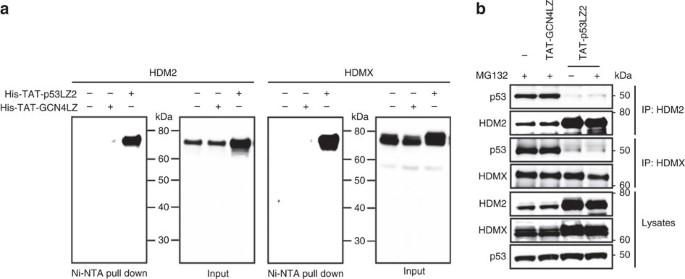Figure 5: TAT-p53LZ2 inhibits direct interactions between p53 and HDM2 or HDMXin situ. (a) MCF7 cells were treated with His-tagged TAT-p53LZ2 or His-tagged TAT-GCN4LZ for 6 h. A total of 10 μM of MG132 was treated for 4 h prior to cell lysis. Cell lysates were subjected to Ni-NTA pull-down followed by immunoblotting with anti-HDM2 or anti-HDMX antibody. (b) Cell lysates were prepared as ina, and then subjected to immunoprecipitation with anti-HDM2 and anti-HDMX antibody followed by immunoblotting with indicated antibodies. Figure 5: TAT-p53LZ2 inhibits direct interactions between p53 and HDM2 or HDMX in situ. ( a ) MCF7 cells were treated with His-tagged TAT-p53LZ2 or His-tagged TAT-GCN4LZ for 6 h. A total of 10 μM of MG132 was treated for 4 h prior to cell lysis. Cell lysates were subjected to Ni-NTA pull-down followed by immunoblotting with anti-HDM2 or anti-HDMX antibody. ( b ) Cell lysates were prepared as in a , and then subjected to immunoprecipitation with anti-HDM2 and anti-HDMX antibody followed by immunoblotting with indicated antibodies. Full size image Reactivation of the p53 pathway in cancer cells by p53LZ2 To examine the effect of p53LZ2 on growth and viability in cancer cells, we treated various exponentially growing cancer cells expressing the wild-type p53 (osteosarcoma SJSA-1, colorectal carcinoma HCT 116, breast carcinoma MCF7 and lung carcinoma A549) or mutant p53 (epidermoid carcinoma A-431 and breast carcinoma MDA-MB-231) with the highly pure recombinant TAT-p53LZ2 produced from E. coli . A dose-dependent anti-proliferative and cytotoxic efficacy of TAT-p53LZ2 accessed by CTG (CellTiter-Glo) assay demonstrated that the cell-permeable TAT-p53LZ2 significantly diminished the cancer cell viability in the wild-type but not mutant p53 cell lines (IC 50 , SJSA-1=3.12 μM, HCT 116=6.13 μM, MCF7=2.20 μM and A549=4.94 μM) ( Fig. 6a ). In addition, we carried out western blot analysis on cancer cell lines incubated with TAT-p53LZ2, TAT-GCN4LZ or Nutlin-3 for 24 h, demonstrating that TAT-p53LZ2 effectively rescued the endogenous p53 and increased the protein expression level of its downstream transcription targets, p21 CIP1/WAF1 and HDM2, in a dose-dependent manner ( Fig. 6b ). On the other hand, p53 phosphorylation, which represents the genotoxic stress and p53 activation in both carcinoma and non-carcinoma by a synthetic compound (for example, doxorubicin), was not detectable in the TAT-p53LZ2-treated cancer cell lines, suggesting the non-genotoxic mechanism of p53 reactivation by delivering exogenously introduced TAT-p53LZ2 into the cancer cells ( Fig. 6c ). Further studies of the real-time quantitative PCR (RT–qPCR) of the wild-type (SJSA-1 and HCT 116) and mutant p53 (A-431 and MDA-MB-231) cancer cell lines revealed that the accumulation of endogenous p53 in cancer cells expressing wild-type p53 by exogenous TAT-p53LZ2 was due to decreased proteasome-mediated p53 degradation rather than increased level of p53 gene expression, while the dose-dependent mRNA induction of three p53 transcriptional targets, p21 CIP1/WAF1 , HDM2 and MIC-1 (macrophage inhibitory cytokine-1), was strongly correlated with elevated p53 levels that restored p53 pathway in cancer cells expressing wild-type p53 ( Fig. 6d ). 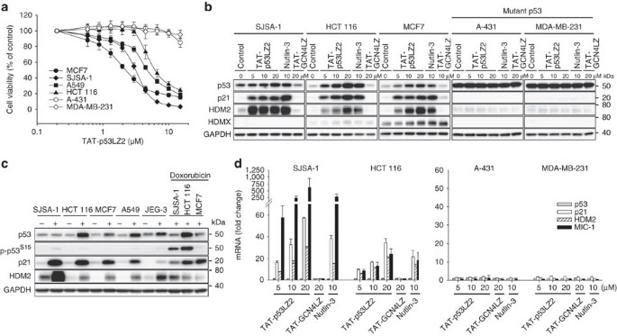Figure 6: TAT-p53LZ2 reactivates p53 signalling pathway in cancer cells expressing wild-type p53. (a) Cell viability of four wild-type p53, SJSA-1, HCT 116, MCF7 and A549, and two mutant p53, A-431 and MDA-MB-231, cancer cell lines was measured by the CellTiter-Glo (CTG) assay after 5-d incubation with TAT-p53LZ2. Data represent the mean±s.d. of three independent experiments. (b) TAT-p53LZ2 stabilizes endogenous p53 and elevates protein levels of p53 targets, p21CIP1/WAF1and HDM2. Three wild-type p53, SJSA-1, HCT 116 and MCF7, and two mutant p53, A-431 and MDA-MB-231, cancer cells were incubated with TAT-p53LZ2, TAT-GCN4LZ or Nutlin-3 and then analysed by western blotting. (c) Exogenously introduced TAT-p53LZ2 does not induce genotoxic response in cancer cells. Cells were incubated with 10 μM of TAT-p53LZ2 or 1 μM of doxorubicin for 24 h and then the phosphorylated p53 at S15 were determined by western blotting. (d) TAT-p53LZ2 but not TAT-GCN4LZ induces p53 target genes in cancer cells bearing WT p53 in a dose-dependent manner. mRNA levels of p53, p21CIP1/WAF1, HDM2 and MIC-1 in cancer cells were determined by the TaqMan RT-qPCR assays. Data represent the mean±s.d. of three independent experiments. Figure 6: TAT-p53LZ2 reactivates p53 signalling pathway in cancer cells expressing wild-type p53. ( a ) Cell viability of four wild-type p53, SJSA-1, HCT 116, MCF7 and A549, and two mutant p53, A-431 and MDA-MB-231, cancer cell lines was measured by the CellTiter-Glo (CTG) assay after 5-d incubation with TAT-p53LZ2. Data represent the mean±s.d. of three independent experiments. ( b ) TAT-p53LZ2 stabilizes endogenous p53 and elevates protein levels of p53 targets, p21 CIP1/WAF1 and HDM2. Three wild-type p53, SJSA-1, HCT 116 and MCF7, and two mutant p53, A-431 and MDA-MB-231, cancer cells were incubated with TAT-p53LZ2, TAT-GCN4LZ or Nutlin-3 and then analysed by western blotting. ( c ) Exogenously introduced TAT-p53LZ2 does not induce genotoxic response in cancer cells. Cells were incubated with 10 μM of TAT-p53LZ2 or 1 μM of doxorubicin for 24 h and then the phosphorylated p53 at S15 were determined by western blotting. ( d ) TAT-p53LZ2 but not TAT-GCN4LZ induces p53 target genes in cancer cells bearing WT p53 in a dose-dependent manner. mRNA levels of p53, p21 CIP1/WAF1 , HDM2 and MIC-1 in cancer cells were determined by the TaqMan RT-qPCR assays. Data represent the mean±s.d. of three independent experiments. Full size image Functional analysis of HDM inhibition by p53LZ2 The consequence of elevated expression levels of the cyclin-dependent kinase (Cdk) inhibitor p21 CIP1/WAF1 mediated by TAT-p53LZ2 is to arrest cell cycle of cancer cells in G 1 and G 2 phases. Treatment of 10 μM of TAT-GCN4LZ, TAT-p53LZ2 or Nutlin-3 for 24 h on various cancer cell lines (wild-type p53: SJSA-1, MCF7, A549 and HCT 116, mutant p53: A-431) demonstrated that EdU (5-ethynyl-2′-deoxyuridine)-labelled cancer cells harbouring wild-type p53 exhibited statistically remarkable cell cycle arrest in G 1 and G 2 –M phases and depletion of S phase population in comparison with other cell line expressing mutant p53 ( Fig. 7a ). Especially, we observed most effective accumulation in G 1 and G 2 –M phases of HCT 116 upon TAT-p53LZ2 treatment (35.8% more in G 1 and 18.7% more in G 2 –M), relative to the other WT p53 cells. Further studies by the quantitative flow cytometry (FACS) analysis also indicated that TAT-p53LZ2 but not TAT-GCN4LZ induces G 1 and G 2 –M cell cycle arrest with a decreased fraction of cells in S phase, confirming that the cell-permeable TAT-p53LZ2 reactivates key machineries of p53 pathway ( Supplementary Fig. 8 ). 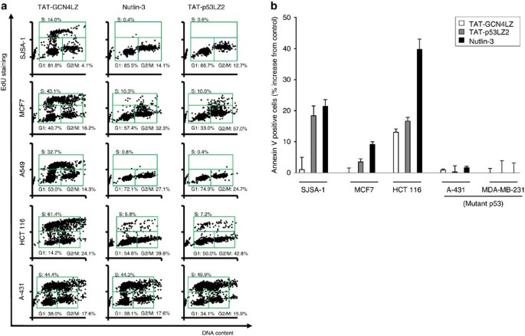Figure 7: TAT-p53LZ2 induces cell cycle arrest and apoptosis in cancer cells. (a) For cell cycle analysis, five cancer cell lines were treated with TAT-p53LZ2, TAT-GCN4LZ or Nutlin-3 for 24 h. Cells were incubated with 10 μM of EdU followed by Alexa fluor 488 labelling and nuclear DNA staining with Hoechst 33342. Cell cycle distribution was calculated from the image analysis and expressed as the percentage of the total population rounded to the full percentage value. (b) Cell lines expressing wild-type or mutant p53 were cultured with 10 μM of TAT-p53LZ2, TAT-GCN4LZ or Nutlin-3 and the percentage of apoptotic cells (±s.d.) was determined by the Annexin V assay after 48 h. Figure 7: TAT-p53LZ2 induces cell cycle arrest and apoptosis in cancer cells. ( a ) For cell cycle analysis, five cancer cell lines were treated with TAT-p53LZ2, TAT-GCN4LZ or Nutlin-3 for 24 h. Cells were incubated with 10 μM of EdU followed by Alexa fluor 488 labelling and nuclear DNA staining with Hoechst 33342. Cell cycle distribution was calculated from the image analysis and expressed as the percentage of the total population rounded to the full percentage value. ( b ) Cell lines expressing wild-type or mutant p53 were cultured with 10 μM of TAT-p53LZ2, TAT-GCN4LZ or Nutlin-3 and the percentage of apoptotic cells (±s.d.) was determined by the Annexin V assay after 48 h. Full size image Next, we investigated the apoptotic activity of TAT-p53LZ2 in cancer cells with wild-type or mutant p53. All cancer cells were treated with 10 μM of Nutlin-3, TAT-GCN4LZ or TAT-p53LZ2 for 48 h, and then analysed by 7-AAD (7-aminoactinomycin D) and Annexin V staining in FACS. After 48 h of incubation with TAT-p53LZ2, 31.4, 22.1 and 18.9% of the cell populations in SJSA-1, MCF7 and HCT 116, respectively, were induced to apoptotic cell death, whereas any cell lines expressing mutant p53 (A-431 and MDA-MB-231) were indistinguishable from the cells treated with TAT-GCN4LZ ( Supplementary Fig. 9 ). Finally, TAT-p53LZ2 was evaluated for its potential antitumour efficacy in the human xenograft model. We chose to perform the study with human colorectal carcinoma HCT 116 (p53+/+). Previous in vitro and/or in vivo studies of HCT 116 with either Nutlin-3 or pMI peptide treatment exhibited a relatively low sensitivity [17] , [39] , encouraging us to tackle this tumour model to assess in vivo potency of TAT-p53LZ2 homodimer, harbouring ~2.5-fold higher affinity against HDMX in vitro compared with WT p53TAD as well as a superb in vitro binding to HDM2. An orally administered Nutlin-3 (200 mg per kg twice a day for 3 weeks) strongly suppressed tumour growth ( P <0.005 versus control; two-sided Student’s t -test), while its intravenous administration was largely ineffective compared with vehicle control ( P =0.37 versus control; two-sided Student’s t -test). In contrast, TAT-p53LZ2 treated intravenously (0.6 mM once a day for 3 weeks) showed notably inhibited tumour growth of HCT 116 xenograft, relative to the vehicle control ( Fig. 8 ). Neither a significant weight loss in the mice nor any abnormalities upon autopsy was observed at the end of the treatment. 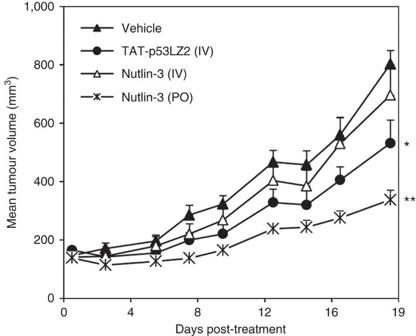Figure 8: TAT-p53LZ2 inhibits tumour growth in a HCT 116 xenograft model. Nude mice (n=8 per group) were implanted subcutaneously (s.c.) with HCT 116 and groups of mice (N=8) received vehicle, TAT-p53LZ2 (0.6 mM) or Nutlin-3 (10 mg kg−1) intravenously once a day for 3 weeks or Nutlin-3 (200 mg kg−1) orally twice a day for 3 weeks. Tumour size was assessed by direct caliper measurement. Data are represented as mean tumour volume ±s.e.m. (*P<0.05, **P<0.005 versus vehicle in two-sided Student’st-test). Figure 8: TAT-p53LZ2 inhibits tumour growth in a HCT 116 xenograft model. Nude mice ( n =8 per group) were implanted subcutaneously (s.c.) with HCT 116 and groups of mice ( N =8) received vehicle, TAT-p53LZ2 (0.6 mM) or Nutlin-3 (10 mg kg −1 ) intravenously once a day for 3 weeks or Nutlin-3 (200 mg kg −1 ) orally twice a day for 3 weeks. Tumour size was assessed by direct caliper measurement. Data are represented as mean tumour volume ±s.e.m. (* P <0.05, ** P <0.005 versus vehicle in two-sided Student’s t -test). Full size image The significant role of the E3 ubiquitin ligase HDM2 and subsequently identified HDMX in regulating tumour suppressor p53 was first revealed by the finding that both HDMs can directly interact with p53 and more significantly HDM2 in turn mediates mono-ubiquitination of p53 in vitro and in vivo [1] , [2] , [11] . A major oncogenic aspect of HDM2 and HDMX is the ability to abolish the transcriptional activity of tumour suppressor p53 (ref. 40 ). Paradoxically, HDM2 itself is the product of the p53 inducible gene, in which it is tightly associated through the auto-regulatory feedback loop aimed at effectively downregulating p53 activity in the absence of stimulus such as hypoxia or DNA damage. Furthermore, the emerging picture in which HDMX plays an independent but also cooperative role with HDM2 in regulating p53 stability makes the regulatory mechanism governing the cellular level of p53 seem more complicated [9] . In addition, recent studies suggest that a dynamic control of both p53 and HDM2 by HAUSP-mediated de-ubiquitination also contribute towards regulating the p53-HDM2 pathway [41] . Therefore, in terms of therapeutic needs in the oncology field, the inactivation of p53 pathway occurred in most human cancers, promotes an awareness of a clear value proposition that restoring wild-type p53 in cancer cells by targeting both HDM2 and HDMX with a potential therapeutic antagonist would be a highly promising strategy for treating cancers. The goal of our studies presented here is to strive towards molecular minimization of p53 while preserving functional activity. Myriad structural and functional versatilities of cellular proteins in biology allow us the way to imitate a particular form and/or function of natural proteins. In our case, the concept of how to properly design structural and functional mimicry performing mostly analogous roles compared with p53, but showing advanced structural and functional integrities was necessary. Accordingly, we came up with biomimetic approach, which is a bio-inspired methodology of creating and constructing new artificial biology systems. Our rational grafting approach has successfully elicited the molecular mimicry of the N-terminal domain of p53 (p53TAD) in the grafted p53LZ2, enforcing the disruption of p53-HDM2 and/or HDMX interaction in vitro and in vivo . The wild-type p53TAD exists with ~11% α-helices in solution with the majority as random coil [25] . Several pioneering concepts suggested that conformation-stabilized polypeptides that capture their bioactive forms have benefits in vitro and in vivo [42] , [43] , [44] , [45] . The p53LZ2 homodimer is stabilized by the LZ motif, through which the close packing of hydrophobic leucine and valine residues between each helices is formed, increasing molecular α-helicity to over 90%. The designed p53LZ2 occupies key accessible positions on HDM2 for the inhibition of protein–protein interaction (PPI). A comparison of in vitro binding characteristics of p53LZ2 shows improvement of its binding to both HDMs compared with WT p53TAD (quantitatively ~3.4- and ~2.5-fold higher affinities to HDM2NTD and HDMXNTD, respectively). Considering the relatively larger binding area of grafted p53LZ2 homodimer in comparison with small synthetic compounds, the binding potency of p53LZ2 may be enhanced further. Moreover, the newly created electrostatic interactions between both proteins, p53LZ2 K3, E6, E20, E22 and HDM2NTD E69, K70, K94, K51, respectively, demonstrated by our structural studies, further reinforce the protein–protein interaction compared with that of WT p53TAD. Given these findings based on our in vitro biochemical and biophysical studies in this early stage of discovery research, we then focused on how to augment the intracellular efficacy of grafted p53LZ2 to eventually overcome a tremendous hurdle of HDM2 and HDMX overexpression in cancer. Numerous efforts have shown that TAT-mediated peptide or protein delivery into cells is capable of modulating various functional activities in vitro and in vivo , including an autophagy-inducing peptide, TAT-beclin-1, and a novel class of neuroprotectant, TAT-NR2B9c (refs 46 , 47 ). TAT-p53LZ2, composed of the HIV-1 TAT protein transduction domain (PTD) attached via (GS) 2 linker to 30 amino acids of each helix of parallel homodimeric p53LZ, as an antagonist to both HDM2 and HDMX, successfully targets endogenous HDM2 and HDMX in cancer cells, preventing p53-HDM interaction, bypassing proteasome-mediated degradation of p53, and thus, leading to the intracellular p53 stabilization. A subsequent activation of the Cdk inhibitor p21 CIP1/WAF1 by p53-signalling cascade in response to exogenous treatment with TAT-p53LZ2 relies on the accumulation of endogenous p53 in cancer cells expressing wild-type but not mutant p53. Unfortunately, the cell-permeable TAT-p53LZ2 is likely more destructive in interfering with p53-HDM2 interaction than with p53-HDMX in our cultured cancer cells, even though TAT-p53LZ2 itself is capable of enhanced binding to HDMX compared with WT p53TAD in vitro . We could not observe statistically significant difference in efficacy between HDM2-overexpressing (for example, SJSA-1) and HDMX-overexpressing (for example, JEG3) p53+/+ cancer cells upon either HDM2-specific Nutlin-3 or TAT-p53LZ2 treatment. Only the anti-proliferative assay of MCF7 upon TAT-p53LZ2 treatment exhibited that the cell viability was reduced by >10% compared with that of Nutlin-3 (IC 50 =3.74 μM for Nutlin-3 versus 2.20 μM for TAT-p53LZ2) ( Supplementary Fig. 10 ). One of possible reasons for this is the elevated level of HDM2 in response to increased levels of wild-type p53 in cells by exogenously introduced TAT-p53LZ2, suggesting that a buildup of the intracellular HDM2 level may compel the equilibrium between both HDMs to move towards p53LZ2-mediated HDM2 homo-dimerization rather than HDMX–HDMX and HDM2–HDMX dimerization, thus decreasing the effective concentration of TAT-p53LZ2 available for HDMX targeting. Our finding that p53 reactivation by antagonizing p53-HDM interaction with exogenously treated TAT-p53LZ2 is capable of inducing not only a cell cycle arrest but also an apoptotic outcome in cancer cells is clearly demonstrated. First, TAT-p53LZ2 and Nutlin-3 but not TAT-GCN4LZ exclusively induced both responses upon pharmacological activation of p53. Second, in contrast to mutant p53, defective in p53-mediated transcriptional activation, cancer cells bearing wild-type p53 were susceptible to both marked changes to regulate cell fate only upon p53 activation by TAT-p53LZ2. Finally, intravenous administration of TAT-p53LZ2 to subcutaneous xenograft HCT 116 tumour model in vivo moderated substantial tumour expansion in mice, compared with the vehicle control, suggesting a possible therapeutic use of TAT-p53LZ2. Future fine-tuned studies will further investigate how strongly the cell-permeable p53LZ2 exhibits its in vivo efficacy. Previously identified high affinity peptide inhibitors (for example, pMI and pDI) disrupting WT p53-HDM interactions are known to possess limited therapeutic scopes by the fact that most of them are less stable and poorly internalized into cells [17] , [48] . It is likely that the largely unstructured nature of those single-chain peptide inhibitors leads to a relative instability in vivo . In addition, these ‘naked’ peptide antagonists in the absence of any particular cell-penetrating moiety that facilitates cellular uptake of fusion partner across the cell membrane is mostly inefficient in cell internalization. Furthermore, stapled p53 peptides, which have to be modified through in vitro chemical synthesis, still have been under development and evaluation processes for therapeutic use [25] , [27] , [49] . Our alternative approach to develop a new molecular entity of HDM dual antagonist, which is readily producible from bacterial expression system, demonstrates that TAT-mediated internalization of highly stabilized α-helical scaffold of p53LZ2 exhibits on-target efficacy in cells. In conclusion, modulation of p53 response with our designed p53LZ2, generated by a rational protein grafting strategy and protein engineering, shows a therapeutic possibility against various cancers and provides a framework to further advance the development of peptide-based drug discovery platform. Protein preparation All constructs were generated by a standard PCR method ( Supplementary Table 2 ). All p53LZ constructs and GCN4LZ were subcloned into NdeI-XhoI of pET21b, BamHI-XhoI of pGEX-4T3 or NdeI-XhoI sites of pDB-HisGST. Full-length (FL) WT p53TAD (residues 1–72) was subcloned into BamHI-XhoI of pGEX-4T3. FL HDM2, HDM2NTD (residues 1–125) and HDMXNTD (residues 1–132) were subcloned into NdeI-XhoI sites of pDB-HisMBP, pET21b or pET28a. Each plasmid was transformed into E. coli BL21(DE3)CodonPlus-RIPL (Agilent Technologies). Protein expression was induced by addition of 0.5 mM of IPTG at OD 600 ~0.8 and then cells were further grown at 18 °C for overnight. For co-purification of p53LZ2-HDM complexes, GST-p53LZ2 mixed with either HDM2NTD or HDMXNTD at 1:2 molar ratio was subjected to GST affinity chromatography followed by anion-exchange chromatography (Mono Q) and size-exclusion chromatography (superdex-75). GST-, MBP- or His-tagged individual proteins were purified by an affinity chromatography, followed by additional purification steps through Mono-Q and gel filtration in the absence or presence of protease cleavage (thrombin or TEV). For all cell-based assays and in vivo studies, the protein storage buffer of TAT-p53LZ2 and TAT-GCN4LZ was exchanged with RPMI-1640 (Gibco). In vitro GST pull-down assay GST, GST-p53LZ1, GST-p53LZ2 or GST-p53LZ3 (3 nmol) was incubated with either His-HDM2NTD or His-HDMXNTD (1:2 molar ratio) for 1 h at 4 °C. A total of 20 μl of glutathione resin was used to pull down GST-fused proteins mixed with HDM. The binding reaction was performed at 4 °C with gentle agitation. The GST-bound resin was washed three times with 500 μl of PBS (pH 7.4) buffer. Proteins were eluted in SDS sample buffer and separated by 12% SDS–PAGE. Multi-angle light scattering analysis The molecular mass of p53LZ2 bound to HDM2NTD or HDMXNTD was determined by the quantitative analysis using MALS. Each sample (5 mg ml −1 , PBS pH 7.4) was injected into a WTC-030S5 column (Wyatt Technology) coupled to 18-angle light scattering detector (DAWN HELEOS II) and a refractive index detector (Optilab T-rEX) (Wyatt Technology). All data were collected at 25 °C (0.5 ml min −1 of flow-rate) and analysed using ASTRA 6 software. Enzyme-linked immunosorbent assay ELISA microtiter plates (Nunc) were coated with 100 μl of MBP-FL HDM2, MBP-HDM2NTD or MBP-HDMXNTD (500 nM) supplemented with 50 mM carbonate/bicarbonate (pH 9.6) for 16 h at 4 °C. After washing the wells with PBS containing 0.05% Tween-20 (PBST buffer), ELISA plates were incubated in blocking buffer (PBS, 0.1% Tween-20 and 3% skim milk) for 2 h at room temperature and then increasing amounts of binding protein (GST or GST-tagged proteins) were added to the wells for 1 h at room temperature. The plates were washed three times with PBST buffer and subsequently incubated with horseradish peroxidase-conjugated anti-GST antibody in blocking buffer (1:2,000) for 1 h. After three times washing, the plates were developed with TMB peroxidase substrate and the absorbance was measured at 450 nm. Isothermal titration calorimetry HDM2NTD, HDMXNTD and p53LZ2 homodimer were extensively dialyzed against PBS (pH 7.4) before titration. The calorimetric titrations were carried out at 18 °C on MicroCal Auto-ITC200 system with 20 consecutive injections of p53LZ2 (0.3 mM, 2 μl each), spaced 200 s apart, into the cell containing either HDM2NTD (0.03 mM) or HDMXNTD (0.025 mM). The raw data were processed with ORIGIN software. The following equations were used to calculate; K D =1 K a −1 ( K D =dissociation constant, K a =association constant), − RT ln K a =Δ G =Δ H − T Δ S (Δ G =free energy change, Δ H =enthalpy change and Δ S =entropy change) Circular dichroism spectroscopy CD spectra and thermal melt analyses of p53LZ2 and GCN4LZ were performed with 20 μM of each protein in PBS (pH 7.4) using a Jasco J-715 spectrometer. The wavelength dependence of [ θ ] was monitored from 190 to 260 nm at 50 nm min −1 speed. All spectra, accumulated three times, were corrected for solvent contributions. The melting profiles were obtained at 220 nm with a heating rate of 2 °C per min. Molecular dynamics simulations MD simulations were performed using GROMACS 4.5.5 coupled with GROMOS-96 53A6 forcefield [50] . The initial structures in this study were generated by the least-square fitting between modified GCN4LZ (PDB ID 2ZTA) and WT p53TAD bound to HDM2 (PDB ID 1YCR) using LSQKAB [51] . Each system was solvated with SPC water and neutralized at the salt concentration of 150 mM by adding appropriate sodium and chloride ions. The initial structures were relaxed through energy minimization followed by two-step equilibrium simulations to relax the solvent and ions while restraints were applied to protein complexes. These calculations were conducted in two phases: 100 ps NVT ( N =moles, V =volume, T =temperature) followed by 100 ps NPT ( N =moles, P =pressure, T =temperature) ensemble dynamics ( T =310 K). MD simulations in production phase were performed in the NPT ensemble for 60 ns with a time step of 2 fs. The long-range electrostatic interactions were treated with the Particle Mesh Ewald (PME) technique while non-bond interactions were truncated with an 1.2-nm cutoff. The MM/PBSA approach was applied to binding energy calculations using GMXAPBS tool [52] , which is a Bash/Perl script to facilitate the interface between GROMACS and APBS [53] . The average of last 15 ns MD simulations (600 frames) was considered to calculate the binding energy and the entropic term was neglected. Structural modelling The initial crystallization trials using a high-throughput nanolitre dispensing robot, the Mosquito (TTP labtech), were performed with hanging drop vapour diffusion method at 18 °C. The optimized p53LZ2 crystals were grown against crystallization buffers containing 0.1 M Tris–HCl (pH 9.0) and 11% ethanol. The drops were set up using 1 μl of the protein solution (3 mg ml −1 in 20 mM Tris HCl (pH 7.4) and 100 mM NaCl) and 1 μl of the reservoir solution. X-ray diffraction data were collected at −170 °C with a single crystal flash-frozen in crystallization buffer supplemented with final 30% glycerol. A native crystal data set was collected at the PAL (Pohang Accelerator Laboratory, South Korea) 5C SB II beamline. Integration, scaling and merging of the diffraction data were performed using the XDS [54] . X-ray structure was determined by molecular replacement method with PHASER [55] using the structure of GCN4LZ (PDB ID 2ZTA) as a search model. Model rebuilding was carried out using COOT [56] , and then modified model was refined by a rigid body protocol followed by energy minimization and simulated-annealing methods in PHENIX [57] . The final structure was assessed with PROCHECK [58] . Comparative protein structure modelling was performed with HADDOCK using crystal structures of p53LZ2 homodimer, HDM2NTD (PDB ID 1YCR) and HDMXNTD (PDB ID 3U15). Active residues were based on solvent accessibility, as well as the structural superposition between p53LZ2 homodimer and WT p53TAD-HDM2NTD (or HDMXNTD) complex. Small-angle X-ray scattering SAXS data collection for p53LZ2-HDM2NTD and p53LZ2-HDMXNTD complexes in PBS pH 7.4 was conducted at the PAL 4C SAXS II beamline (0.675 Å). All SAXS measurements were done in triplicate exposures at 18 °C and the scattering from the buffer alone were subtracted from the solution scattering data of each protein sample. Exposure times were typically 10 min for individual measurements. The controlled sample-to-detector distance (1–4 m) was applied to collect the complete data set of both complexes. All data were processed and analysed using the ATSAS software suite including PRIMUS, GNOM and CRYSOL [59] , [60] , [61] . Ab initio SAXS envelopes for both p53LZ2-HDM complexes were calculated using GASBOR [37] . Immunoprecipitation and pull-down For immunoprecipitation, MCF7 cells were solubilized in lysis buffer containing protease inhibitor and phosphatase inhibitor (Roche). Cell lysates were incubated with indicated antibody at 4 °C overnight. The antigen–antibody complex was added to protein A/G resins (Thermo) and incubated for 2 h at 4 °C. The resins were collected by centrifugation, and then washed three times with lysis buffer and twice with buffer A supplemented with 20 mM Tris–HCl pH 7.4, 150 mM NaCl and 0.1 M EDTA. For Ni-NTA pull-down, the cell lysates were incubated with Ni-NTA beads for 2 h at 4 °C and then washed three times with buffer B containing 20 mM Tris–HCl pH 7.4, 150 mM NaCl, 1 mM EDTA, 0.2% Tween-20 and 20 mM imidazole. Bound proteins were eluted by 0.2% SDS and separated by SDS–PAGE, followed by immunoblotting with the appropriate antibodies. Cell assays and western blots All human cell lines were purchased from the American Type Culture Collection (ATCC). Cells were cultured in the indicated media supplemented with 10% fetal bovine serum (Gibco) and 1% Zell Shield (Minerva biolabs) at 37 °C in 5% CO 2 . For cell viability assay, cells (1 × 10 3 –2 × 10 3 cells) were seeded in 96-well plates and treated with TAT-p53LZ2 or TAT-GCN4LZ at the indicated concentrations for 5 days. Cell viability assays were performed in triplicate and assessed with CellTiter-Glo (Promega) by using EnVision Multilabel Reader (PerkinElmer). For western blotting, cells were grown in six-well plates (4 × 10 5 cells per well) and lysed in 0.1–0.2 ml of lysis buffer (cOmplete lysis kit, Roche). The following antibodies were used; p53 (Santa Cruz sc-126, 1:200 dilution), HDMX (Santa Cruz sc-374147, 1:100 dilution), GAPDH (Santa Cruz sc-25778, 1:200 dilution), p21 (Cell Signaling no. 2947, 1:500 dilution), p-p53 (Cell Signaling no. 9284, 1:1,000 dilution), HDM2 (Abcam ab-16895, 1:50 dilution), anti-mouse IgG-HRP (Cell Signaling no. 7076, 1:2,000 dilution) and anti-rabbit IgG-HRP (Cell Signaling no. 7074, 1:2,000 dilution). Uncropped versions of representative western blots used in the current study are shown in Supplementary Figs 11 and 12 . Quantitative RT–PCR Total RNA was extracted using RNeasy Mini Kit (Qiagen) from cells treated with vehicle, TAT-p53LZ2, TAT-GCN4LZ or Nutlin-3 (Sigma) at 37 °C for 24 h. cDNA was prepared from total RNA using the high-capacity RNA-to-cDNA kit (Applied Biosystems). RT-qPCR was performed by using TaqMan Gene Expression Master Mix (Applied Biosystems) and gene-specific primer/probe set (Applied Biosystems, TP53 (Hs00153349_m1), HDM2 (Hs00242813_m1), p21 ( CDKN1A ) (Hs00355782_m1), MIC-1 ( GDF15 ) (Hs00171132_m1) and GAPDH (Hs99999905_m1)) on a LightCycler 480 (Roche). Data were analysed with the LightCycler 480 software (Roche) determining the threshold cycle ( C t ). Relative quantities of mRNA were calculated using comparative cycle threshold method after normalization to GAPDH . Cell cycle arrest and apoptotic assays For cell cycle analysis, SJSA-1, MCF7, A549, HCT 116 and A-431 cells were plated in a μ-bottom 96-well plate (ibidi GmbH). After 24 h, all cells were incubated with 10 μM of TAT-p53LZ2, TAT-GCN4LZ or Nutlin-3 for 24 h. For EdU uptake, cells were incubated with 10 μM of EdU for 1.5 h. EdU labelling was performed using Click-reaction with Alexa fluor 488 in EdU staining kit (C10350, Invitrogen). Nuclear DNA was stained with Hoechst 33342. Cell imaging was conducted using Incell Analyzer 6000 (GE healthcare). Captured images were analysed using MTA (multi-target analysis) module of Incell communicator (image analysis software, GE healthcare) to obtain parameters and cell cycle population. Nuclear integrated intensity of Hoechst 33342 and EdU as parameters were used to plot cell population. For apoptotic cell measurement by Annexin V-PE and 7-AAD staining, SJSA-1, MCF7, HCT 116, A-431 and MDA-MB-231 cells were incubated with 10 μM of TAT-p53LZ2, TAT-GCNLZ or Nutlin-3 (Sigma). After 48 h, cells were harvested and resuspended in 0.2 ml of binding buffer and then stained with Annexin V-PE/7-AAD (BD bioscience) for 15 min at room temperature, followed by FACS analysis. Growth inhibition of human HCT 116 xenograft model All animals were dosed and monitored according to guidelines from the Institutional Animal Care and Use Committee (IACUC) at ChemOn Inc. Female BALB/c nude mice (6–8 weeks old) were purchased from Japan SLC Inc (Shizuoka, Japan). Mice were injected (right flank) subcutaneously with HCT 116 cells (3 × 10 5 cells per mouse; suspended in 100 ml of PBS mixed with 100 ml of BD Matrigel). Once tumours reached a mean volume of ~150 mm 3 , all tumour-bearing animals were randomized into four study groups according to tumour sizes. Mice were treated via tail vein with vehicle control (RPMI-1640) or TAT-p53LZ2. Nutin-3 was treated via either intravenously (dissolved in 5% DMSO and 5% dextrose) or orally (dissolved in 2% HPMC and 0.2% Tween-80). Animals were monitored and tumours were measured every 2–3 days. The length ( L ) and width ( W ) of the tumour mass were measured, and the tumour volume (TV) was calculated as: TV=( L × W 2 ) × 2 −1 . Accession codes: The atomic coordinate of p53LZ2 has been deposited in the Protein Data Bank under the accession code 4OWI . How to cite this article: Lee, J.-H. et al. Protein grafting of p53TAD onto a leucine zipper scaffold generates a potent HDM dual inhibitor. Nat. Commun. 5:3814 doi: 10.1038/ncomms4814 (2014).